Sustainable biochar to mitigate global climate change Production of biochar (the carbon (C)-rich solid formed by pyrolysis of biomass) and its storage in soils have been suggested as a means of abating climate change by sequestering carbon, while simultaneously providing energy and increasing crop yields. Substantial uncertainties exist, however, regarding the impact, capacity and sustainability of biochar at the global level. In this paper we estimate the maximum sustainable technical potential of biochar to mitigate climate change. Annual net emissions of carbon dioxide (CO 2 ), methane and nitrous oxide could be reduced by a maximum of 1.8 Pg CO 2 -C equivalent (CO 2 -C e ) per year (12% of current anthropogenic CO 2 -C e emissions; 1 Pg=1 Gt), and total net emissions over the course of a century by 130 Pg CO 2 -C e , without endangering food security, habitat or soil conservation. Biochar has a larger climate-change mitigation potential than combustion of the same sustainably procured biomass for bioenergy, except when fertile soils are amended while coal is the fuel being offset. Since 2000, anthropogenic carbon dioxide (CO 2 ) emissions have risen by more than 3% annually [1] , putting Earth's ecosystems on a trajectory towards rapid climate change that is both dangerous and irreversible [2] . To change this trajectory, a timely and ambitious programme of mitigation measures is needed. Several studies have shown that, to stabilize global mean surface temperature, cumulative anthropogenic greenhouse-gas (GHG) emissions must be kept below a maximum upper limit, thus indicating that future net anthropogenic emissions must approach zero [2] , [3] , [4] , [5] , [6] . If humanity oversteps this threshold of maximum safe cumulative emissions (a limit that may already have been exceeded [7] ), no amount of emissions reduction will return the climate to within safe bounds. Mitigation strategies that draw down excess CO 2 from the atmosphere would then assume an importance greater than an equivalent reduction in emissions. Production of biochar, in combination with its storage in soils, has been suggested as one possible means of reducing the atmospheric CO 2 concentration (refs [8] , [9] , [10] , [11] , [12] , [13] and see also Supplementary Note for a history of the concept and etymology of the term). Biochar's climate-mitigation potential stems primarily from its highly recalcitrant nature [14] , [15] , [16] , which slows the rate at which photosynthetically fixed carbon (C) is returned to the atmosphere. In addition, biochar yields several potential co-benefits. It is a source of renewable bioenergy; it can improve agricultural productivity, particularly in low-fertility and degraded soils where it can be especially useful to the world's poorest farmers; it reduces the losses of nutrients and agricultural chemicals in run-off; it can improve the water-holding capacity of soils; and it is producible from biomass waste [17] , [18] . Of the possible strategies to remove CO 2 from the atmosphere, biochar is notable, if not unique, in this regard. Biochar can be produced at scales ranging from large industrial facilities down to the individual farm [19] , and even at the domestic level [20] , making it applicable to a variety of socioeconomic situations. Various pyrolysis technologies are commercially available that yield different proportions of biochar and bioenergy products, such as bio-oil and syngas. The gaseous bioenergy products are typically used to generate electricity; the bio-oil may be used directly for low-grade heating applications and, potentially, as a diesel substitute after suitable treatment [21] . Pyrolysis processes are classified into two major types, fast and slow, which refer to the speed at which the biomass is altered. Fast pyrolysis, with biomass residence times of a few seconds at most, generates more bio-oil and less biochar than slow pyrolysis, for which biomass residence times can range from hours to days. 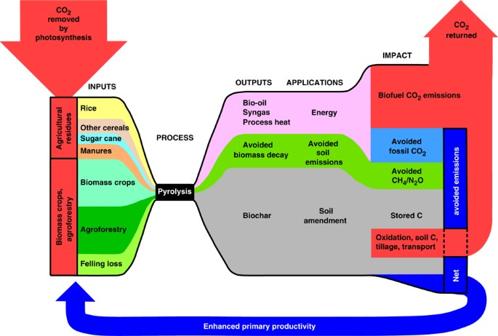Figure 1: Overview of the sustainable biochar concept. The figure shows inputs, process, outputs, applications and impacts on global climate. Within each of these categories, the relative proportions of the components are approximated by the height/width of the coloured fields. CO2is removed from the atmosphere by photosynthesis to yield biomass. A sustainable fraction of the total biomass produced each year, such as agricultural residues, biomass crops and agroforestry products, is converted by pyrolysis to yield bio-oil, syngas and process heat, together with a solid product, biochar, which is a recalcitrant form of carbon and suitable as a soil amendment. The bio-oil and syngas are subsequently combusted to yield energy and CO2. This energy and the process heat are used to offset fossil carbon emissions, whereas the biochar stores carbon for a significantly longer period than would have occurred if the original biomass had been left to decay. In addition to fossil energy offsets and carbon storage, some emissions of methane and nitrous oxide are avoided by preventing biomass decay (seeSupplementary Table S5for example) and by amending soils with biochar. Additionally, the removal of CO2by photosynthesis is enhanced by biochar amendments to previously infertile soils, thereby providing a positive feedback. CO2is returned to the atmosphere directly through combustion of bio-oil and syngas, through the slow decay of biochar in soils, and through the use of machinery to transport biomass to the pyrolysis facility, to transport biochar from the same facility to its disposal site and to incorporate biochar into the soil. In contrast to bioenergy, in which all CO2that is fixed in the biomass by photosynthesis is returned to the atmosphere quickly as fossil carbon emissions are offset, biochar has the potential for even greater impact on climate through its enhancement of the productivity of infertile soils and its effects on soil GHG fluxes. The sustainable-biochar concept is summarized in Figure 1 . CO 2 is removed from the atmosphere by photosynthesis. Sustainably procured crop residues, manures, biomass crops, timber and forestry residues, and green waste are pyrolysed by modern technology to yield bio-oil, syngas, process heat and biochar. As a result of pyrolysis, immediate decay of these biomass inputs is avoided. The outputs of the pyrolysis process serve to provide energy, avoid emissions of GHGs such as methane (CH 4 ) and nitrous oxide (N 2 O), and amend agricultural soils and pastures. The bioenergy is used to offset fossil-fuel emissions, while returning about half of the C fixed by photosynthesis to the atmosphere. In addition to the GHG emissions avoided by preventing decay of biomass inputs, soil emissions of GHGs are also decreased by biochar amendment to soils. The biochar stores carbon in a recalcitrant form that can increase soil water- and nutrient-holding capacities, which typically result in increased plant growth. This enhanced productivity is a positive feedback that further enhances the amount of CO 2 removed from the atmosphere. Slow decay of biochar in soils, together with tillage and transport activities, also returns a small amount of CO 2 to the atmosphere. A schematic of the model used to calculate the magnitudes of these processes is shown as Supplementary Figure S1 . Figure 1: Overview of the sustainable biochar concept. The figure shows inputs, process, outputs, applications and impacts on global climate. Within each of these categories, the relative proportions of the components are approximated by the height/width of the coloured fields. CO 2 is removed from the atmosphere by photosynthesis to yield biomass. A sustainable fraction of the total biomass produced each year, such as agricultural residues, biomass crops and agroforestry products, is converted by pyrolysis to yield bio-oil, syngas and process heat, together with a solid product, biochar, which is a recalcitrant form of carbon and suitable as a soil amendment. The bio-oil and syngas are subsequently combusted to yield energy and CO 2 . This energy and the process heat are used to offset fossil carbon emissions, whereas the biochar stores carbon for a significantly longer period than would have occurred if the original biomass had been left to decay. In addition to fossil energy offsets and carbon storage, some emissions of methane and nitrous oxide are avoided by preventing biomass decay (see Supplementary Table S5 for example) and by amending soils with biochar. Additionally, the removal of CO 2 by photosynthesis is enhanced by biochar amendments to previously infertile soils, thereby providing a positive feedback. CO 2 is returned to the atmosphere directly through combustion of bio-oil and syngas, through the slow decay of biochar in soils, and through the use of machinery to transport biomass to the pyrolysis facility, to transport biochar from the same facility to its disposal site and to incorporate biochar into the soil. In contrast to bioenergy, in which all CO 2 that is fixed in the biomass by photosynthesis is returned to the atmosphere quickly as fossil carbon emissions are offset, biochar has the potential for even greater impact on climate through its enhancement of the productivity of infertile soils and its effects on soil GHG fluxes. Full size image Even under the most zealous investment programme, biochar production will ultimately be limited by the rate at which biomass can be extracted and pyrolysed without causing harm to the biosphere or to human welfare. Globally, human activity is responsible for the appropriation of 16 Pg C per year from the biosphere, which corresponds to 24% of potential terrestrial net primary productivity (NPP) [22] . Higher rates of appropriation will increase pressure on global ecosystems, exacerbating a situation that is already unsustainable [23] . The main aim of this study is to provide an estimate of the theoretical upper limit, under current conditions, to the climate-change mitigation potential of biochar when implemented in a sustainable manner. This limit, which we term the maximum sustainable technical potential (MSTP), represents what can be achieved when the portion of the global biomass resource that can be harvested sustainably (that is, without endangering food security, habitat or soil conservation) is converted to biochar by modern high-yield, low-emission, pyrolysis methods. The fraction of the MSTP that is actually realized will depend on a number of socioeconomic factors, including the extent of government incentives and the relative emphasis placed on energy production relative to climate-change mitigation. Aside from assuming a maximum rate of capital investment that is consistent with that estimated to be required for climate-change mitigation [24] , this study does not take into account any economic, social or cultural barriers that might further limit the adoption of biochar technology. Our analysis shows that sustainable global implementation of biochar can potentially offset a maximum of 12% of current anthropogenic CO 2 -C equivalent (CO 2 -C e ) emissions (that is, 1.8 Pg CO 2 -C e per year of the 15.4 Pg CO 2 -C e emitted annually), and that over the course of a century, the total net offset from biochar would be 130 Pg CO 2 -C e . We also show that conversion of all sustainably obtained biomass to maximize bioenergy, rather than biochar, production can offset a maximum of 10% of the current anthropogenic CO 2 -C e emissions. The relative climate-mitigation potentials of biochar and bioenergy depend on the fertility of the soil amended and the C intensity of the fuel being offset, as well as the type of biomass. Locations at which the soil fertility is high and coal is the fuel being offset are best suited for bioenergy production. The climate-mitigation potential of biochar (with combined energy production) is higher for all other situations. Sustainable biomass-feedstock availability To ensure that our estimates represent a sustainable approach, we use a stringent set of criteria to assess potential feedstock availability for biochar production. Of primary importance is the conversion of land to generate feedstock. In addition to its negative effects on ecosystem conservation, land clearance to provide feedstock may also release carbon stored in soils and biomass, leading to unacceptably high carbon-payback times before any net reduction in atmospheric CO 2 is achieved (ref. 25 , Supplementary Methods and Supplementary Fig. S2 ). For example, we find that a land-use change carbon debt greater than 22 Mg C ha −1 (an amount that would be exceeded by conversion of temperate grassland to annual crops [25] ) will result in a carbon-payback time that is greater than 10 years. Clearance of rainforests to provide land for biomass-crop production leads to carbon payback times in excess of 50 years. Where rainforest on peatland is converted to biomass-crop production, carbon-payback times may be in the order of 325 years. We therefore assume that no land clearance will be used to provide biomass feedstock, nor do we include conversion of agricultural land from food to biomass-crop production as a sustainable source of feedstock, both because of the negative consequences for food security and because it may indirectly induce land clearance elsewhere [26] . Some dedicated biomass-crop production on abandoned, degraded agricultural soil has been included in this study as this will not adversely affect food security [27] and can improve biodiversity [28] , [29] . We further assume that extraction rates of agricultural and forestry residues are sufficiently low to preclude soil erosion or loss of soil function, and that no industrially treated waste biomass posing a risk of soil contamination will be used. Other constraints on biochar production methods arise because emissions of CH 4 , N 2 O, soot or volatile organic compounds combined with low biochar yields (for example, from traditional charcoal kilns or smouldering slash piles) may negate some or all of the carbon-sequestration benefits, cause excessive carbon-payback times or be detrimental to health. Therefore, we do not consider any biochar production systems that rely on such technologies, and restrict our analysis to systems in which modern, high-yield, low-emission pyrolysis technology can feasibly be used to produce high-quality biochar. Within these constraints, we derived a biomass-availability scenario for our estimate of MSTP, as well as two additional scenarios, Alpha and Beta, which represent lower demands on global biomass resources ( Table 1 ). Attainment of the MSTP would require substantial alteration to global biomass management, but would not endanger food security, habitat or soil conservation. The Alpha scenario restricts biomass availability to residues and wastes available using current technology and practices, together with a moderate amount of agroforestry and biomass cropping. All three scenarios represent fairly ambitious projects, and require progressively greater levels of political intervention to promote greater adoption of sustainable land-use practices and increase the quantity of uncontaminated organic wastes available for pyrolysis. We do not consider any scenarios that are not ambitious in this study, as the intention is to investigate whether biochar could make a substantial contribution to climate-change mitigation—an aspiration that certainly will not be accomplished by half-hearted measures. The range of mitigation results reported thus refers only to the scenarios considered and does not encompass the full range of less-effective outcomes corresponding to varying levels of inaction. The scenarios are based on current biomass availability ( Supplementary Methods and Supplementary Tables S1 and S2 ), the composition and energy contents of different types of biomass and the biochar derived from each ( Supplementary Tables S3 and S4 ), and the rate of adoption of biochar technology ( Supplementary Fig. S3 ). How this biomass resource base changes over the course of 100 years will depend on the potential effects of changing climate, atmospheric CO 2 , sea level, land use, agricultural practices, technology, population, diet and economic development. Some of these factors may increase biomass availability and some may decrease it. A full assessment of the wide range of possible future scenarios within plausible ranges of these factors remains outside the scope of this study. Table 1 Annual globally sustainable biomass feedstock availability. Full size table Avoided GHG emissions Results for the three scenarios are expressed below as a range from the Alpha scenario first to the MSTP last. The model predicts that maximum avoided emissions of 1.0–1.8 Pg CO 2 -C e per year are approached by mid-century and that, after a century, the cumulative avoided emissions are 66–130 Pg CO 2 -C e ( Fig. 2 ). Half of the avoided emissions are due to the net carbon sequestered as biochar, 30% to replacement of fossil-fuel energy by pyrolysis energy and 20% to avoided emissions of CH 4 and N 2 O. Cumulative and annual avoided emissions for the individual gases CO 2 , CH 4 and N 2 O are given in Supplementary Figures S4 , S5 and S6 . 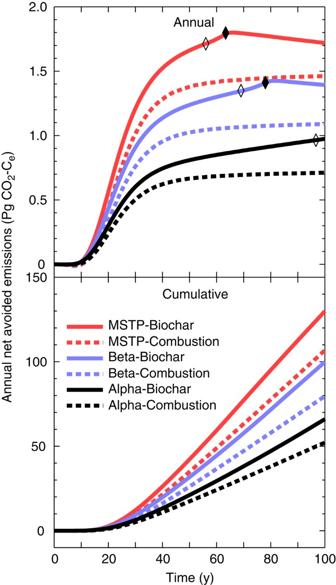Figure 2: Net avoided GHG emissions. The avoided emissions are attributable to sustainable biochar production or biomass combustion over 100 years, relative to the current use of biomass. Results are shown for the three model scenarios, with those for sustainable biochar represented by solid lines and for biomass combustion by dashed lines. The top panel shows annual avoided emissions; the bottom panel, cumulative avoided emissions. Diamonds indicate transition period when biochar capacity of the top 15 cm of soil fills up and alternative disposal options are needed. Figure 2: Net avoided GHG emissions. The avoided emissions are attributable to sustainable biochar production or biomass combustion over 100 years, relative to the current use of biomass. Results are shown for the three model scenarios, with those for sustainable biochar represented by solid lines and for biomass combustion by dashed lines. The top panel shows annual avoided emissions; the bottom panel, cumulative avoided emissions. Diamonds indicate transition period when biochar capacity of the top 15 cm of soil fills up and alternative disposal options are needed. 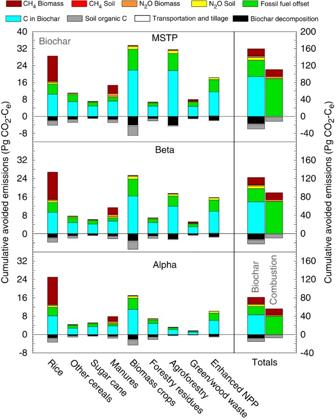Figure 3: Breakdown of cumulative avoided GHG emissions (Pg CO2-Ce) from sustainable biochar production. The data are for the three model scenarios over 100 years by feedstock and factor. The left side of the figure displays results for each of eight feedstock types and the additional biomass residues that are attributed to NPP increases from biochar amendments; the right side displays total results by scenario for both biochar (left column) and biomass combustion (right column). For each column, the total emission-avoiding and emission-generating contributions are given, respectively, by the height of the columns above and below the zero line. The net avoided emissions are calculated as the difference between these two values. Within each column, the portion of its contribution caused by each of six emission-avoiding mechanisms and three emission-generating mechanisms is shown by a different colour. These mechanisms (from top to bottom within each column) are (1) avoided CH4from biomass decay, (2) increased CH4oxidation by soil biochar, (3) avoided N2O from biomass decay, (4) avoided N2O caused by soil biochar, (5) fossil fuel offsets from pyrolysis energy production, (6) avoided CO2emissions from carbon stored as biochar, (7) decreased carbon stored as soil organic matter caused by diversion of biomass to biochar, (8) CO2emissions from transportation and tillage activities and (9) CO2emissions from decomposition of biochar in soil. Full size image A detailed breakdown of the sources of cumulative avoided GHG emissions over 100 years is given in Figure 3 . The two most important factors contributing to the avoided emissions from biochar are carbon stored as biochar in soil (43–94 Pg CO 2 -C e ) and fossil-fuel offsets from coproduction of energy (18–39 Pg CO 2 -C e ). Figure 3: Breakdown of cumulative avoided GHG emissions (Pg CO 2 -C e ) from sustainable biochar production. The data are for the three model scenarios over 100 years by feedstock and factor. The left side of the figure displays results for each of eight feedstock types and the additional biomass residues that are attributed to NPP increases from biochar amendments; the right side displays total results by scenario for both biochar (left column) and biomass combustion (right column). For each column, the total emission-avoiding and emission-generating contributions are given, respectively, by the height of the columns above and below the zero line. The net avoided emissions are calculated as the difference between these two values. Within each column, the portion of its contribution caused by each of six emission-avoiding mechanisms and three emission-generating mechanisms is shown by a different colour. These mechanisms (from top to bottom within each column) are (1) avoided CH 4 from biomass decay, (2) increased CH 4 oxidation by soil biochar, (3) avoided N 2 O from biomass decay, (4) avoided N 2 O caused by soil biochar, (5) fossil fuel offsets from pyrolysis energy production, (6) avoided CO 2 emissions from carbon stored as biochar, (7) decreased carbon stored as soil organic matter caused by diversion of biomass to biochar, (8) CO 2 emissions from transportation and tillage activities and (9) CO 2 emissions from decomposition of biochar in soil. Full size image Of the beneficial feedbacks, the largest is due to avoided CH 4 emissions from biomass decomposition (14–17 Pg CO 2 -C e ), predominantly arising from the diversion of rice straw from paddy fields (see Supplementary Table S5 for estimate of the mean CH 4 emission factor). The next largest positive feedbacks, in order of decreasing magnitude, arise from biochar-enhanced NPP on cropland, which contributes 9–16 Pg CO 2 -C e to the net avoided emissions (if these increased crop residues are converted to biochar), followed by reductions in soil N 2 O emissions (4.0–6.2 Pg CO 2 -C e ), avoided N 2 O emissions during biomass decomposition (1.8–3.3 Pg CO 2 -C e ) and enhanced CH 4 oxidation by dry soils (0.44–0.8 Pg CO 2 -C e ). Of the adverse feedbacks, biochar decomposition is the largest (8–17 Pg CO 2 -C e ), followed by loss of soil organic carbon due to diversion of biomass from soil into biochar production (6–10 Pg CO 2 -C e ), and transport (1.3–1.9 Pg CO 2 -C e , see Supplementary Fig. S7 ). Contributions to the overall GHG budget from tillage (0.03–0.044 Pg CO 2 -C e ) and reduced N-fertilizer production (0.2–0.3 Pg CO 2 -C e ) are negligible (although their financial costs may not be). The relative importance of all these factors to the GHG budget varies considerably among feedstocks. Notably, rice residues, green waste and manure achieve the highest ratios of avoided CO 2 -C e emissions per unit of biomass-carbon (1.2–1.1, 0.9 and 0.8 CO 2 -C e /C, respectively) because of the benefits of avoided CH 4 emissions. Sensitivity and Monte Carlo analyses Sensitivity and Monte Carlo analyses with respect to reasonable values of key variables were used to estimate the uncertainty of the model results; they suggest areas in which future research is most needed and provide guidance on how biochar production systems might be optimized ( Fig. 4 ). 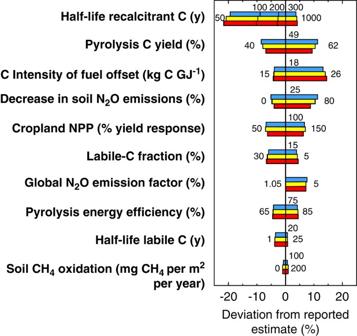Figure 4: Sensitivity of the model to key variables. Sensitivity is expressed as a percentage deviation from the reported value of cumulative net avoided GHG emissions over 100 years for each scenario. Top (blue), middle (yellow) and bottom (red) bars for each variable correspond to Alpha, Beta and MSTP scenarios. Minimum and maximum values for each variable are at the ends of the bars (with additional sensitivities to recalcitrant carbon half-life of 100 and 200 years shown); baseline values of the key variables used in this study correspond to 0% deviation. See alsoSupplementary Table S7. Figure 4: Sensitivity of the model to key variables. Sensitivity is expressed as a percentage deviation from the reported value of cumulative net avoided GHG emissions over 100 years for each scenario. Top (blue), middle (yellow) and bottom (red) bars for each variable correspond to Alpha, Beta and MSTP scenarios. Minimum and maximum values for each variable are at the ends of the bars (with additional sensitivities to recalcitrant carbon half-life of 100 and 200 years shown); baseline values of the key variables used in this study correspond to 0% deviation. See also Supplementary Table S7 . Full size image The strongest sensitivity is to the half-life of the recalcitrant fraction of biochar (see also Supplementary Table S6 ). Net avoided GHG emissions vary by −22% to +4% from that obtained using the baseline assumption of 300 years. However, most of this variation occurs for half-life <100 years, in which range we find (in agreement with previous work [30] ) that sensitivity to this factor is high. Conversely, for a more realistic half-life of the recalcitrant fraction (>100 years), sensitivity to this factor is low because biochar can be produced much more rapidly than it decays. As currently available data suggest that the half-life of biochar's recalcitrant fraction in soil is in the millennial range (see Supplementary Methods , Supplementary Table S6 and refs [8] , [15] , [16] , [31] 8, 15, 16, 31), the contribution of its decay to the net GHG balance over centennial timescales is likely to be small. The next largest sensitivity is to the pyrolysis carbon yield (−9% to +11%), indicating the importance of engineering to optimize for high yields of biochar rather than for energy production. This will be constrained, however, by the sensitivity to the labile fraction of the biochar (−7% to +4%), which indicates the importance of optimizing for production of recalcitrant biochar rather than for higher yields of lower-quality biochar. After carbon yield, the next largest sensitivity is to the carbon intensity of the fuel offset by pyrolysis energy production, with net avoided emissions varying by −4% from the baseline assumption when natural gas is the fuel being offset and by +15% when coal is offset. Varying the impact of biochar amendment on soil N 2 O emissions from zero to the largest reported reduction (80%; ref. 32 ) produces a sensitivity of −4% to +11%. Further variability in the impact of biochar on N 2 O emissions arises from adjusting the fraction of biomass-N that (if left to decompose) would be converted to N 2 O-N, from the Intergovernmental Panel on Climate Change default values assumed in this study up to the higher rate of 5% suggested by more recent work [33] , [34] . This would increase the net avoided GHG emissions by up to 8%. Uncertainty in the response of crop yields to biochar amendment results in estimated range of −6% to +7% in the impact of enhanced NPP of cropland on net avoided GHG emissions. Sensitivities to the pyrolysis energy efficiency (±5%), to the half-life of the biochar's labile fraction (−4% to +1%) and to its impact on soil CH 4 oxidation (± 1%) are small. The net effect of covariance of the above factors was assessed using the Monte Carlo analysis ( n =1,000, Supplementary Table S7 ). Despite limited data on the decomposition rate of biochar in soils and the effects of biochar additions on soil GHG fluxes, sensitivity within realistic ranges of these parameters is small, resulting in an estimated uncertainty of ±8 to 10% (±1 s.d.) in the cumulative avoided GHG emissions for the three scenarios. Comparison of biochar and bioenergy approaches The mitigation impact of the renewable energy obtained from both biochar production and biomass combustion depends on the carbon intensity (that is, the mass of carbon emitted per unit of total energy produced) of the offset energy sources [11] . At our baseline carbon intensity (17.5 kg C GJ −1 ; see Methods section), the model predicts that, on an average, the mitigation impact of biochar is 27–22% (14–23 Pg CO 2 -C e ) larger than the 52–107 Pg CO 2 -C e predicted if the same sustainably procured biomass were combusted to extract the maximum amount of energy ( Fig. 2 ). This advantage of biochar over bioenergy is largely attributable to the beneficial feedbacks from enhanced crop yields and soil GHG fluxes ( Fig. 3 , Supplementary Fig. S8 ). Because the principal contribution of biomass combustion to avoided GHG emissions is the replacement of fossil fuels ( Fig. 3 ), the bioenergy approach shows a considerably higher sensitivity to carbon intensity than does biochar ( Fig. 5 ). The carbon intensity of offset energy varies from near-zero for renewable and nuclear energy to 26 kg C GJ −1 for coal combustion [35] . Mean cumulative avoided emissions from biochar and biomass combustion are equal in our scenarios when the carbon intensity of offset energy is 26–24 kg C GJ −1 ( Fig. 5 ). In the MSTP scenario, this corresponds to an energy mix to which coal combustion contributes about 80%, whereas in the Alpha scenario, the mean mitigation benefit of biochar remains higher than that of bioenergy, even when 100% coal is offset. The cumulative avoided emissions from both strategies decrease as the carbon intensity of the offset energy mix decreases, but the rate of decrease for biomass combustion is 2.5–2.7 times greater than that for biochar. As expected, the cumulative avoided emissions for biomass combustion are essentially zero when the carbon intensity of the energy mix is also zero. In contrast, the cumulative avoided emissions for biochar are still substantial at 48–91 Pg CO 2 -C e . 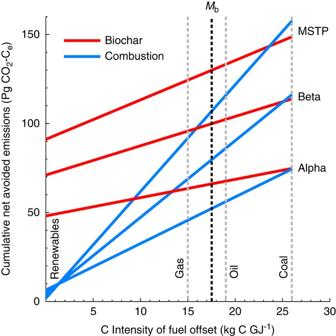Figure 5: Cumulative mitigation potential (100 years) of biochar and biomass combustion as a function of carbon intensity of the type of energy being offset. The black vertical dashed line labelledMbon the upperxaxis refers to the carbon intensity of the baseline energy mix assumed in this study. Grey vertical dashed lines at 15, 19 and 26 kg C GJ−1denote the carbon intensity of natural gas, oil and coal, respectively. The carbon intensity of renewable forms of energy is close to 0 kg C GJ−1. Figure 5: Cumulative mitigation potential (100 years) of biochar and biomass combustion as a function of carbon intensity of the type of energy being offset. The black vertical dashed line labelled M b on the upper x axis refers to the carbon intensity of the baseline energy mix assumed in this study. Grey vertical dashed lines at 15, 19 and 26 kg C GJ −1 denote the carbon intensity of natural gas, oil and coal, respectively. The carbon intensity of renewable forms of energy is close to 0 kg C GJ −1 . Full size image Given that much of the increased climate mitigation from biochar relative to biomass combustion stems from the beneficial feedbacks of adding biochar to soil, and that these feedbacks will be greatest on the least fertile soils, the relative mitigation potentials will vary regionally with soil type (see Supplementary Methods , Supplementary Fig. S9 and Supplementary Tables S8–S11 for an account of how these feedbacks are calculated). 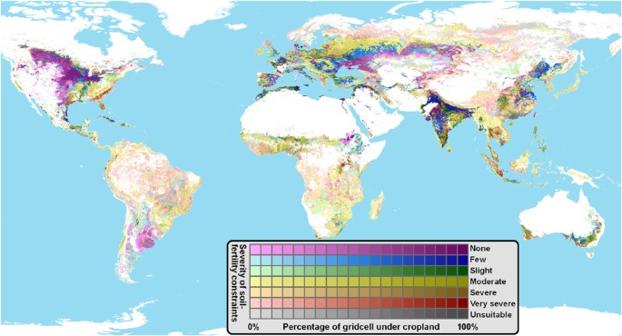Figure 6: Soil-fertility constraints to cropland productivity (5′ resolution). Soil fertility is indicated by hue, whereas the percentage of the gridcell currently being used as cropland is indicated by colour saturation (with white indicating the absence of cropland in a grid cell). The distribution of soils of varying fertility on global cropland is shown in Figure 6 . Globally, 0.31 Gha of soils with no fertility constraints are in use as cropland, as well as 0.29 Gha of cropland with few fertility constraints, 0.21 Gha with slight constraints, 0.32 Gha with moderate constraints, 0.18 Gha with severe constraints, 0.13 Gha with very severe constraints and 0.09 Gha of cropland on soils categorized as unsuitable for crop production. The amount of biomass produced in soils of different fertilities is shown in Supplementary Table S12 . 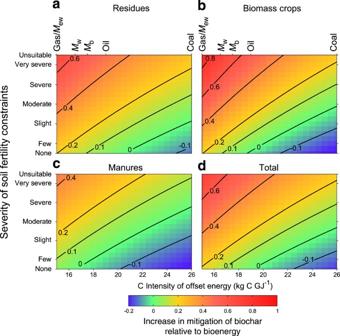Figure 7: Cumulative mitigation potential of biochar relative to bioenergy. The mitigation potential is reported as a function of both soil fertility and carbon intensity of the type of energy being offset (in the MSTP scenario). PointsMew,MwandMbon the upperxaxis refer to the carbon intensity of the current world electricity mix, the current world primary energy mix and the baseline energy mix assumed in our scenarios, respectively. Carbon intensity values for natural gas, oil and coal are also indicated. The relative mitigation is calculated as cumulative avoided emissions for biochar minus those for bioenergy, expressed as a fraction of the avoided emissions for bioenergy (for example, a value of 0.1 indicates that the cumulative mitigation impact of biochar is 10% greater than that of bioenergy, a value of −0.1 indicates that it is 10% lower and a value of zero indicates that they have the same mitigation impact). The soil-fertility classifications marked on the vertical axis correspond to the soil categories mapped inFigure. 6. Panela(Residues) includes agricultural and forestry residues, together with green waste, as biomass inputs; Panelb(Biomass crops) includes both dedicated biomass crops and agroforestry products as biomass inputs. Panelc(Manures), includes bovine, pig and poultry manure as biomass inputs. Paneld(Total) includes all sources of biomass inputs in the proportions assumed in our model. An analogous figure for the Alpha scenario is shown asSupplementary Figure S10. Figure 7 shows how the climate mitigation from biochar varies relative to biomass combustion when both soil fertility and the carbon intensity of energy offsets are considered. The relative benefit of producing biochar compared with biomass combustion is greatest when biochar is added to marginal lands and the energy produced by pyrolysis is used to offset natural gas, renewable or nuclear energy. When biochar is added to the most infertile cropland to offset the current global primary energy mix ( M w ), which has a carbon intensity of 16.5 kg C GJ −1 , the relative benefit from biochar is as much as 79–64% greater than that from bioenergy ( Fig. 7 , Supplementary Fig. S10 ). This net benefit diminishes as more coal is offset and as biochar is added to soils with higher fertility. Nevertheless, with the exception of those geographical regions having both naturally high soil fertility and good prospects for offsetting coal emissions (in which bioenergy yields up to 16–22% greater mitigation impact than biochar), biochar shows a greater climate-mitigation potential than bioenergy. The relative benefit of producing biochar compared with bioenergy is greatest when biomass crops are used as feedstocks ( Fig. 7b ), because avoided CH 4 emissions from the use of manure, green waste and rice residues occur regardless of whether these other feedstocks are used for energy or biochar. Figure 6: Soil-fertility constraints to cropland productivity (5′ resolution). Soil fertility is indicated by hue, whereas the percentage of the gridcell currently being used as cropland is indicated by colour saturation (with white indicating the absence of cropland in a grid cell). Full size image Figure 7: Cumulative mitigation potential of biochar relative to bioenergy. The mitigation potential is reported as a function of both soil fertility and carbon intensity of the type of energy being offset (in the MSTP scenario). Points M ew , M w and M b on the upper x axis refer to the carbon intensity of the current world electricity mix, the current world primary energy mix and the baseline energy mix assumed in our scenarios, respectively. Carbon intensity values for natural gas, oil and coal are also indicated. The relative mitigation is calculated as cumulative avoided emissions for biochar minus those for bioenergy, expressed as a fraction of the avoided emissions for bioenergy (for example, a value of 0.1 indicates that the cumulative mitigation impact of biochar is 10% greater than that of bioenergy, a value of −0.1 indicates that it is 10% lower and a value of zero indicates that they have the same mitigation impact). The soil-fertility classifications marked on the vertical axis correspond to the soil categories mapped in Figure. 6 . Panel a (Residues) includes agricultural and forestry residues, together with green waste, as biomass inputs; Panel b (Biomass crops) includes both dedicated biomass crops and agroforestry products as biomass inputs. Panel c (Manures), includes bovine, pig and poultry manure as biomass inputs. Panel d (Total) includes all sources of biomass inputs in the proportions assumed in our model. An analogous figure for the Alpha scenario is shown as Supplementary Figure S10 . Full size image Our analysis demonstrates that sustainable biochar production (with addition to soils) has the technical potential to make a substantial contribution to mitigating climate change. Maximum avoided emissions of the order of 1.8 Pg CO 2 -C e annually, and of 130 Pg CO 2 -C e over the course of a century, are possible at current levels of feedstock availability, while preserving biodiversity, ecosystem stability and food security. The biochar scenarios described here, with their very high levels of biomass utilization, are not compatible with simultaneous implementation of an ambitious biomass energy strategy. The opportunity cost of this forgone energy resource must be taken into account in an economic comparison of the two strategies. However, in terms of their potentials for climate-change mitigation, the mitigation impact of biochar is about one-fourth larger, on an average, than that obtained if the same biomass were combusted for energy. Regional deviations from this average are large because of differences in soil fertility and available biomass. Our model predicts that the relative climate-mitigation benefit of biochar compared with bioenergy is greatest in regions in which poor soils growing biomass crops can benefit most from biochar additions. In contrast, biomass combustion leads to a greater climate-mitigation impact in regions with fertile soils where coal combustion can be effectively offset by biomass energy production. The global climate-mitigation potential achievable from the use of terrestrial biomass may thus be maximized by a mixed strategy favouring bioenergy in those regions with fertile soils where coal emissions can be offset, and biochar elsewhere. Nevertheless, we have included biochar production in fertile, coal-intensive regions in our scenarios because other potential benefits of biochar, such as its potential for more efficient use of water and crop nutrients [36] , [37] , [38] , may favour its use even in such regions. We emphasize that the results presented here assume that future biochar production follows strict sustainability criteria. Land-use changes that incur high carbon debts and biochar production using technologies with poorly controlled emissions lead to both large reductions in avoided emissions and excessively long carbon-payback times, during which net emissions are increased before any net reduction is observed. Biochar production and use, therefore, must be guided by well-founded and well-enforced sustainability protocols if its potential for mitigating climate change is to be realized. Overall approach A model (BGRAM version 1.1) to calculate the net avoided GHG emissions attributable to sustainable biochar production as a function of time was developed and applied to the three scenarios. This model includes the effects of feedstock procurement, transport, pyrolysis, energy production, soil incorporation, soil GHG flux, soil fertility and fertilizer use (see also Supplementary Table S13 ), and biomass and biochar decomposition (see also Supplementary Fig. S11 ). The net avoided GHG emissions due to biochar were calculated as the difference between the CO 2 -equivalent emissions from biochar production and those that would have occurred as the biomass decomposed by other means had it not been converted to biochar. All emissions (actual or avoided) were calculated with time dependency. Wherever possible, conservative assumptions were used to provide a high degree of confidence that our results represent a conservative estimate of the avoided GHG emissions achievable in each scenario. A detailed account of both the model and the three scenarios is given in Supplementary Methods . Sustainability criteria Biochar can be produced sustainably or unsustainably. Our criteria for sustainable biochar production require that biomass procured from agricultural and silvicultural residues be extracted at a rate and in a manner that does not cause soil erosion or soil degradation; crop residues currently in use as animal fodder not be used as biochar feedstock; minimal carbon debt be incurred from land-use change or use of feedstocks with a long life expectancy; no new lands be converted into biomass production and no agricultural land be taken out of food production; no biomass wastes that have a high probability of contamination, which would be detrimental to agricultural soils, be used; and biomass crop production be limited to production on abandoned agricultural land that has not subsequently been converted to pasture, forest or other uses. We further require that biochar be manufactured using modern technology that eliminates soot, CH 4 and N 2 O emissions while recovering some of the energy released during the pyrolysis process for subsequent use. Greenhouse gases We consider three GHGs in this analysis: CO 2 , CH 4 and N 2 O (see Supplementary Table S14 for a summary of estimated global warming potentials for these GHGs). Although the different atmospheric lifetimes of these gases ensure that there is no equivalence among them in any strict sense, we nevertheless adopt the common practice of normalizing each gas to a 'CO 2 -C equivalent' using the estimated radiative forcing produced by the emission of each gas, integrated over a 100-year period following emission, using Intergovernmental Panel on Climate Change 100-year global warming potentials [39] of 23 for CH 4 and 296 for N 2 O. Comparison with bioenergy To compare the net avoided GHG emissions stemming from biochar with those from bioenergy production, we apply the same model and sustainability criteria, but assume complete combustion to liberate the maximum possible energy, rather than slow pyrolysis, as the conversion technology. Soil application and fertility classification Maximum biochar application to the top 0.15 m of agricultural soils was assumed to be 50 Mg C ha −1 . It was assumed that only 20% of pasture soils will receive these application rates because of constraints from terrain, accessibility, fire and wind. See Supplementary Methods and Supplementary Figure S12 . Soil-fertility classifications were taken from ref. 40 . These were combined with a 5-minute resolution map of global cropland distribution [41] to produce a global map of cropland, categorized by the severity of soil-fertility constraints ( Fig. 6 ). Carbon intensity of fuel offsets The baseline carbon intensity of the fuel offsets ( M b ) used here is 17.5 kg C GJ −1 . The current world primary-energy mix ( M w ) has a carbon intensity of 16.5 kg C GJ −1 and the current world electricity-generation mix ( M ew ) has a carbon intensity of 15 kg C GJ −1 (ref. 42 ). See Supplementary Methods for the derivation of these carbon intensities. Technology adoption rate The rate at which installed biochar production capacity approaches its maximum is constrained by simple economic considerations. Data for estimated capital costs are shown in Supplementary Table S15 . These are implemented in the model using a Gompertz curve ( Supplementary Methods ). The model allows for a lead time of 5 years, during which little plant capacity is commissioned. Slow-to-moderate investment for the remainder of the first decade and rapid adoption over the following three decades at a rate of capital investment consistent with the 2% of global gross domestic product that Lord Stern estimates to be required for climate-change mitigation [24] culminate in near-maximal biochar production rates after a total of four decades. Net avoided GHG emissions over the first decade are negligible, because of a combination of initially slow adoption and carbon-debt payback. How to cite this article: Woolf, D. et al . Sustainable biochar to mitigate global climate change. Nat. Commun. 1:56 doi: 10.1038/ncomms1053 (2010).